One-dimensional self-confinement promotes polymorph selection in large-area organic semiconductor thin films A crystal’s structure has significant impact on its resulting biological, physical, optical and electronic properties. In organic electronics, 6,13(bis-triisopropylsilylethynyl)pentacene (TIPS-pentacene), a small-molecule organic semiconductor, adopts metastable polymorphs possessing significantly faster charge transport than the equilibrium crystal when deposited using the solution-shearing method. Here, we use a combination of high-speed polarized optical microscopy, in situ microbeam grazing incidence wide-angle X-ray-scattering and molecular simulations to understand the mechanism behind formation of metastable TIPS-pentacene polymorphs. We observe that thin-film crystallization occurs first at the air–solution interface, and nanoscale vertical spatial confinement of the solution results in formation of metastable polymorphs, a one-dimensional and large-area analogy to crystallization of polymorphs in nanoporous matrices. We demonstrate that metastable polymorphism can be tuned with unprecedented control and produced over large areas by either varying physical confinement conditions or by tuning energetic conditions during crystallization through use of solvent molecules of various sizes. Achieving a desired crystal structure is of great importance to many technologically important materials used in fields such as organic electronics, microelectronics, photonics as well as pharmaceutical and food industries [1] , [2] , [3] , [4] , [5] . For example, the crystal structure of an edible ingredient can influence its taste and texture; in the pharmaceutical industry, different crystal polymorphs of the same drug can have drastically different dissolution rates, bioavailability and chemical stability [2] , [6] . In the field of organic electronics, small aromatic molecules are widely used as the organic semiconductors (OSCs) for thin-film transistors (TFTs) to fabricate a variety of flexible, transparent and bendable electronics [7] , [8] , [9] , [10] , [11] , [12] . The OSC chemical structure, together with π–π stacking and van der Waals intermolecular interactions, collectively determine the molecular packing structure. The electronic coupling between adjacent molecules and the intrinsic charge transport rate, measured by its charge carrier mobility in organic TFT (OTFT) devices, are governed by molecular packing structure [13] . Various polymorphs of a single OSC may exist, with each polymorph exhibiting different carrier mobility owing to differences in their respective π–π stacking structures [14] , [15] . We have previously observed that crystalline thin films of 6,13-(bis-triisopropylsilylethynyl)pentacene (TIPS-pentacene) can be processed into different polymorphs by the solution-shearing deposition method [5] , [16] . The molecular packing was shown to be finely tuned by forming metastable polymorphs with various degrees of structural deviation from the equilibrium polymorph. The lattice was found to expand along the (010) direction while contracting along the (101) direction with increasing solution-shearing speed [5] . This deviation from the equilibrium structure has been shown to result in a shorter distance along certain crystallographic directions between the adjacent TIPS-pentacene molecules, and thus led to stronger intermolecular electronic coupling, yielding faster charge transport [5] . Using a related approach, known as Fluid Enhanced Crystal Engineering (FLUENCE), single crystalline thin films of these polymorphs were fabricated with mobilities as high as 11 cm 2 V −1 s −1 (ref. 16 ). To date, only a small number of OSC thin films have been reported to show mobilities approaching 10 cm 2 V −1 s −1 (refs 17 , 18 , 19 ). Therefore, understanding the formation mechanism of high-performance polymorphs when deposited by large-area solution-processing methods such as solution shearing is imperative to develop a general strategy to further improve charge carrier transport in OSCs. Furthermore, such insight may also provide useful information to other fields where polymorphism critically impacts material properties. A wide range of solution-processing methods has previously been reported to deposit OSC thin films with mixed results. For example, the rather straightforward approach of drop casting usually results in non-uniform films [20] . Inkjet printing, spray-coating and spin coating have also been used to prepare high-mobility OTFTs from a variety of OSCs [21] , [22] , [23] , [24] . These methods generally yield little preferential crystallographic orientation in the plane of the generated thin films without additional patterning processes. By contrast, methods such as zone casting, dip coating, flow coating, knife coating and doctor blading have been shown to produce thin films with preferential in-plane crystallographic orientation over large areas [25] , [26] , [27] . The solution-shearing method was recently proposed as a large-area coating method capable of producing preferential in-plane crystallographic alignment [5] , [28] . This approach entails a top shearing plate forming a well-defined gap that drags the OSC solution across a heated bottom substrate while keeping the bulk of the solution sandwiched between the plate and the substrate, with only the evaporation front of the solution exposed to air [29] . Using the solution-shearing method, we have produced various polymorphs of TIPS-pentacene, a feature reported only in few other thin-film solution-processing methods [5] , [16] , [30] . Direct investigation of the formation of OSC polymorphs is challenging because thin-film crystallization in typical solution-shearing conditions ranges in duration from tens of milliseconds to several seconds and the growth takes place both vertically and laterally [28] . In situ X-ray diffraction has been previously used to provide insight to a variety of solution deposition processes, for example, the formation of OSCs films by drop casting, the formation of the photoactive layer in organic photovoltaics using spin coating and knife coating, the film formation of dip-coated nanoparticles and the formation of microstructures of collagen [31] , [32] , [33] , [34] , [35] , [36] . We have combined high-speed in situ microbeam grazing incidence wide-angle X-ray scattering (μGIWAXS) with high-speed in situ polarized optical microscopy (POM) to investigate the growth sequence of TIPS-pentacene polymorphs during solution shearing [28] . Here we find that crystallization is initiated at the liquid–air interface, thereby self-confining the solution first in a thin liquid film, and then between a crust at the surface of the solution and the substrate. We demonstrate this one-dimensional (1D) self-confinement of the crystallization front between the surface crust and the substrate is responsible for the polymorph selection ability of the solution-shearing process. Careful selection of molar volume of the solvent and surface tension also show unprecedented control of polymorphism, and this effect is explored with the help of molecular simulations. The 1D self-confinement process we report here is analogous to three dimensional (3D) nanoscale confinement in porous media used by the pharmaceutical industry to select polymorphism by using the size-dependent polymorphism of organic crystals [37] , [38] . The solution-shearing method has the added advantage of producing selected polymorphs over large areas, potentially in a roll-to-roll manner, without the requirement of a porous medium. The continuity of polymorph thin films is a critical requirement for the fabrication of large-area electronics and circuitry, and may also have applications in the area of pharmaceuticals and beyond. In situ characterization of solution shearing of TIPS-pentacene films In situ time-resolved measurements of thin-film growth during solution shearing were performed at beamline D1 at the Cornell High Energy Synchrotron Source (CHESS) using μGIWAXS [28] , [39] . An X-ray microbeam focused to a 15 × 15 μm 2 spot is required, as the evaporation front (meniscus) can be as small as 100 μm wide ( Supplementary Movie 1 ). The microbeam was focused by using a single-bounce X-ray capillary [39] . The sample was mounted on the temperature-controlled solution-shearing setup, and thin-film formation was viewed with an optical microscope during solution shearing [28] . The evaporation front can move at a speed of several millimetres per second, thus requiring μGIWAXS data collection at a rate of up to 100 Hz or 10 ms per frame, which is the maximum frame rate of the Dectris Pilatus 100 k detector used in this study. The high-speed POM measurements were collected on an identical solution-shearing setup in the King Abdullah University of Science and Technology (KAUST), with a high-speed colour camera capable of a collection rate of up to 10,000 Hz using a linearly polarized light source. Recently, Headrick and colleagues [30] reported stresses and buckling occurred in thin films of TIPS-pentacene during hollow capillary writing. The time resolution in the study was approximately 0.3 s. However, successful investigation of the crystallization process in the presence of the laterally moving crystal growth front requires the use of high-speed microbeam X-ray-scattering techniques with millisecond time resolution [39] . In Fig. 1a , we show a schematic of the in situ solution-shearing setup at CHESS. The reciprocal space region probed by the fast two-dimensional (2D) X-ray detector is highlighted in Fig. 1b . As diffraction peak intensity is correlated to the number of coherent planes, it can be used to qualitatively monitor the onset, evolution and end of the crystallization process during solution shearing. The position of the diffraction peak is correlated to the unit cell geometry and reveals which polymorphs are formed. Close inspection of the diffraction peak positions has revealed that the equilibrium polymorph is produced exclusively at shearing speeds <0.4 mm s −1 , whereas the coexistence of metastable polymorphs is observed at greater shearing speeds ( T =90 °C and 8 mg ml −1 in toluene) [5] . In Supplementary Fig. 1a,b , we trace the temporal evolution of the (0–11) diffraction peak intensity during solution shearing. The duration of the crystallization process decreases rapidly with increasing shearing speed from 1 s or longer at 0.8 mm s −1 to ~50 ms at 2.8 mm s −1 , indicating a drastically increasing rate of crystallization. However, for shearing speeds above 2.8 mm s −1 (up to 12 mm s −1 ), the rate of crystallization appears to remain comparatively unchanged ( Supplementary Fig. 1b ). 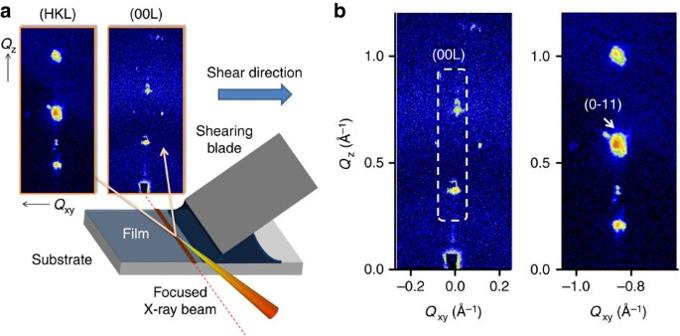Figure 1: Conceptual representation of thein situsolution-shearing system. (a) The focused X-ray microbeam (~15 μm) impinges on the drying front of the OSC solution as the shearing blade moves from left to right and perpendicular to the microbeam. The time series captures crystallization as the OSC solution dries and an OSC crystalline thin-film is formed. (b) Scattering regions captured by the high-speed GIWAXS detector for a representative solution sheared TIPS-pentacene thin film. The different scattering peaks of interest are labelled. Figure 1: Conceptual representation of the in situ solution-shearing system. ( a ) The focused X-ray microbeam (~15 μm) impinges on the drying front of the OSC solution as the shearing blade moves from left to right and perpendicular to the microbeam. The time series captures crystallization as the OSC solution dries and an OSC crystalline thin-film is formed. ( b ) Scattering regions captured by the high-speed GIWAXS detector for a representative solution sheared TIPS-pentacene thin film. The different scattering peaks of interest are labelled. Full size image Time evolution of metastable polymorphs Monitoring both the intensity and the position of the (0–11) diffraction peak during in situ μGIWAXS measurements can help us to better understand the mechanism of formation of metastable polymorphs of TIPS-pentacene. For films sheared at 0.8 mm s −1 ( T =50 °C and 8 mg ml −1 in toluene), we detect a weak (0–11) diffraction signal at first corresponding to the equilibrium crystal structure between 0 and 120 ms, followed by the appearance at ~130 ms of a shifted (0–11) diffraction peak, indicating the formation of the metastable polymorph ( Fig. 2a ; Supplementary Movie 1 ). In Fig. 2b , we trace the time evolution of the integrated intensities of the equilibrium and metastable (0–11) Bragg peaks. It is clearly observed that the equilibrium polymorph is formed first, followed by formation of the metastable polymorph. The equilibrium peak intensity does not decrease, indicating that the two polymorphs coexist rather than transform into one another. In situ POM images taken under the same shearing conditions visually revealed formation of a ribbon-like crystalline film well before 130 ms, that is, in the regime where only the equilibrium polymorph is detected. The images reveal no further change in the appearance of the film in the regime where the metastable polymorph appeared (>130 ms, Supplementary Movie 2 ), indicating that the metastable polymorph does not simply form next to the equilibrium polymorph. The evidence suggests that the two polymorphs are vertically stacked ( Supplementary Note 1 ). We have included other conditions of shearing wherein the equilibrium peak-formed first-is followed by metastable polymorph formation. The time evolution of the (0–11) Bragg peak intensity can be seen in Supplementary Figs 2 and 3 , and in Supplementary Movies 3 and 4 . Supplementary Movie 4 in particular shows the formation of a prominent secondary (0–11) Bragg peak. 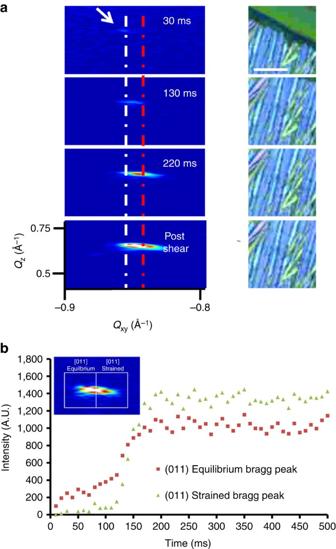Figure 2: Temporal evolution of TIPS-pentacene thin films. (a) Temporal evolution of the equilibrium polymorph followed by formation of the metastable polymorph during thin-film growth, for TIPS-pentacene thin films sheared at 0.8 mm s−1, 8 mg ml−1and 50 °C. The white arrow marks the location of the equilibrium polymorph. The red line marks the strained polymorph that is formed after 130 ms. The correspondingin situhigh-speed POM snapshots reveal no change in the appearance of crystals, implying that the metastable crystallites leading to increase of the (0–11) Bragg peak intensity grow commensurately with the equilibrium crystallites formed near the surface of the film. The scale bar in POM images is 50 μm in length. (b) Integrated intensities of the equilibrium and metastable components of the (0–11) Bragg peak. The inset shows the areas chosen for integration. Figure 2: Temporal evolution of TIPS-pentacene thin films. ( a ) Temporal evolution of the equilibrium polymorph followed by formation of the metastable polymorph during thin-film growth, for TIPS-pentacene thin films sheared at 0.8 mm s −1 , 8 mg ml −1 and 50 °C. The white arrow marks the location of the equilibrium polymorph. The red line marks the strained polymorph that is formed after 130 ms. The corresponding in situ high-speed POM snapshots reveal no change in the appearance of crystals, implying that the metastable crystallites leading to increase of the (0–11) Bragg peak intensity grow commensurately with the equilibrium crystallites formed near the surface of the film. The scale bar in POM images is 50 μm in length. ( b ) Integrated intensities of the equilibrium and metastable components of the (0–11) Bragg peak. The inset shows the areas chosen for integration. Full size image Vertical spatial evolution of metastable polymorphs From the sequence of crystallization, we know that the equilibrium phase forms first, but this sequence does not prove conclusively that crystallization begins mainly at the liquid–air interface, even though concentration is highest here owing to solvent evaporation. We have therefore performed static μGIWAXS measurements at different angles of incidence in order to establish the structural depth profile of the TIPS-pentacene polymorphs. Below the critical angle, only the structure of the top few nanometres of the TIPS-pentacene film are probed by evanescent X-rays, whereas at higher incidence angles the X-ray beam probes the full depth of the thin film. In Fig. 3a,b , we show the intensity distribution of the equilibrium and the metastable polymorphs within the (0–11) Bragg peak for the incidence angles of 0.04° and 0.14°, respectively. The intensity ratio of the metastable peak to the equilibrium peak increases at the higher incidence angle, indicating that the metastable polymorph is buried beneath the equilibrium polymorph. This qualitative depth profile confirms the presence of the metastable polymorph sandwiched between the surface equilibrium layer and the substrate ( Supplementary Fig. 4 ). The time-resolved and static μGIWAXS measurements therefore both point to the polymorph formation sequence illustrated in Fig. 3c . 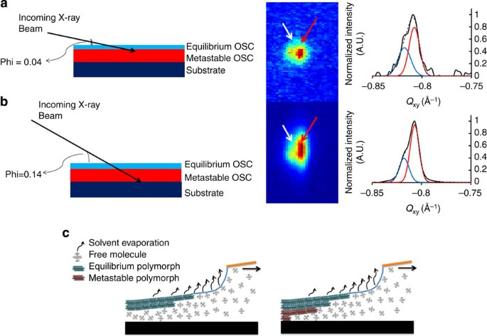Figure 3: Depth profiling studies of TIPS-pentacene thin films. (a,b) Depth profiling of the metastable and equilibrium components of the (0–11) Bragg peak of TIPS-pentacene thin films sheared at 0.8 mm s−1, 8 mg ml−1and 50 °C. (a) The incidence angle of 0.04° preferentially samples the top few nanometres of the film. (b) The incidence angle of 0.14° samples the entire film. The white arrow marks the equilibrium peak, whereas the red arrow marks the metastable peak. The blue and red curves show the Gaussian deconvolution of the integrated peak intensity. The blue curve shows the intensity of the equilibrium peak position and the red curve shows the intensity of the metastable peak position. The ratio of the metastable (0–11) Bragg peak to the equilibrium (0–11) Bragg peak increases, implying that the metastable polymorph preferentially grows as crystallites approach the substrate. (c) Conceptual illustration of how crystal growth proceeds during solution shearing. The equilibrium polymorph (blue unit cells) first forms at the solution–air interface and begins to grow downwards towards the substrate. The metastable polymorph (red unit cells) forms soon after. This may be because of the confinement of the OSC solution in between the equilibrium layer and the substrate. Figure 3: Depth profiling studies of TIPS-pentacene thin films. ( a , b ) Depth profiling of the metastable and equilibrium components of the (0–11) Bragg peak of TIPS-pentacene thin films sheared at 0.8 mm s −1 , 8 mg ml −1 and 50 °C. ( a ) The incidence angle of 0.04° preferentially samples the top few nanometres of the film. ( b ) The incidence angle of 0.14° samples the entire film. The white arrow marks the equilibrium peak, whereas the red arrow marks the metastable peak. The blue and red curves show the Gaussian deconvolution of the integrated peak intensity. The blue curve shows the intensity of the equilibrium peak position and the red curve shows the intensity of the metastable peak position. The ratio of the metastable (0–11) Bragg peak to the equilibrium (0–11) Bragg peak increases, implying that the metastable polymorph preferentially grows as crystallites approach the substrate. ( c ) Conceptual illustration of how crystal growth proceeds during solution shearing. The equilibrium polymorph (blue unit cells) first forms at the solution–air interface and begins to grow downwards towards the substrate. The metastable polymorph (red unit cells) forms soon after. This may be because of the confinement of the OSC solution in between the equilibrium layer and the substrate. Full size image Tuning metastable polymorph by vertical spatial confinement To verify the self-confinement hypothesis, we examine the polymorphism of thin films prepared with different thicknesses (16±4, 40±9 and 68±13 nm) obtained by varying the solution concentration (4, 8 and 16 mg ml −1 , respectively). All other process conditions being kept constant, including the shearing speed (2.8 mm s −1 ) and the substrate temperature (90 °C), the concentration difference is expected to yield different self-confinement conditions. In Fig. 4a , we show in situ POM images of the meniscus region, indicating significant lengthening of the meniscus with decreasing concentration of TIPS-pentacene solution. This is because of the concentration requirements of crystallization that result in a longer solvent evaporation period and consequently a longer and much thinner solution film near the crystallization front. The thinned solution confines the crystallization front in a narrower gap between the air–solvent interface and the substrate ( Supplementary Figs 5 and 6 ). In Fig. 4b , we plot the (0–11) diffraction peak for the three films grown in varying self-confinement conditions. The position of the (0–11) diffraction peak for the film formed in conditions of minimum confinement (68 nm, 16 mg ml −1 ) corresponds to the equilibrium polymorph and is marked with a dashed white line that acts as a guide to the eye. As confinement conditions are increased by decreasing the starting concentration and the thickness of the film while maintaining the process temperature and shearing speed constant, the position of the (0–11) diffraction peak shifts gradually away from that of the equilibrium polymorph, indicating metastable polymorph selection ( Fig. 4b ), just as one would expect on the basis of the spatial confinement hypothesis [37] . 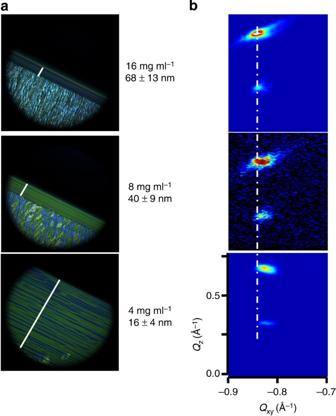Figure 4: Polymorph formation as a function of starting OSC solution concentrations. (a)In situPOM of solution sheared TIPS-pentacene films in toluene at 90 °C and 2.8 mm s−1. The meniscus length (white line) increases as TIPS-pentacene concentration decreases, implying that the TIPS-pentacene crystal nucleation occurs when the meniscus is thinner. The field of view is 1 mm. (b) The (0–11) Bragg peak shifts away from the equilibrium peak position with decreasing solution concentration. The dashed white line marks the position of the equilibrium phase (0–11) Bragg peak and is present to guide the eye. Figure 4: Polymorph formation as a function of starting OSC solution concentrations. ( a ) In situ POM of solution sheared TIPS-pentacene films in toluene at 90 °C and 2.8 mm s −1 . The meniscus length (white line) increases as TIPS-pentacene concentration decreases, implying that the TIPS-pentacene crystal nucleation occurs when the meniscus is thinner. The field of view is 1 mm. ( b ) The (0–11) Bragg peak shifts away from the equilibrium peak position with decreasing solution concentration. The dashed white line marks the position of the equilibrium phase (0–11) Bragg peak and is present to guide the eye. Full size image Tuning metastable polymorph formation by solvent selection The influence of spatial confinement was further investigated by replacing toluene with other solvents while keeping the concentration (8 mg ml −1 ) and shearing speed (0.8 mm s −1 ) fixed ( Fig. 5a,b ). Importantly, we have attempted to maintain the evaporation conditions constant through careful control of solution-shearing temperature. Close-ups of the (011) and (101) diffraction peaks from TIPS-pentacene thin films cast from different solvents reveal that solvents with a larger molar volume further enhanced the formation of metastable polymorphs, whereas solvents with a small molar volume negated the effects of spatial confinement almost entirely. It therefore appears that vertical spatial confinement is not alone in mediating polymorphism; the choice of solvent offers an entirely new process parameter that can either promote metastable polymorphism or prevent it altogether. 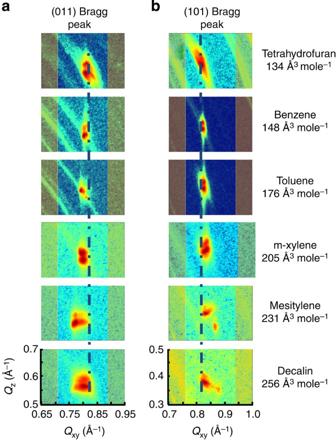Figure 5: Solvent volume confinement effect on TIPS-pentacene thin films. (a) Shift in the (011) Bragg peaks from the equilibrium position as a function of solvent molar volume. (b) Shift in the (101) Bragg peaks from the equilibrium position as a function of solvent molar volume.Increasing the size of solvent molecules (while holding the solvent evaporation rate constant by adjusting the process temperature) leads to more prominence of the metastable polymorphs. The blue lines indicate the equilibriumQxyposition of the (101) and (011) Bragg peaks. All TIPS-pentacene thin films were sheared at a speed of 0.8 mm s−1and 8 mg ml−1. Figure 5: Solvent volume confinement effect on TIPS-pentacene thin films. ( a ) Shift in the (011) Bragg peaks from the equilibrium position as a function of solvent molar volume. ( b ) Shift in the (101) Bragg peaks from the equilibrium position as a function of solvent molar volume.Increasing the size of solvent molecules (while holding the solvent evaporation rate constant by adjusting the process temperature) leads to more prominence of the metastable polymorphs. The blue lines indicate the equilibrium Q xy position of the (101) and (011) Bragg peaks. All TIPS-pentacene thin films were sheared at a speed of 0.8 mm s −1 and 8 mg ml −1 . Full size image Crystallographic texture is very important to small-molecule OTFTs, where most of the successful systems are characterized by the formation of lamellar sheets with 2D in-plane π-stacking, whereby all crystallites can take part in charge transport. Li et al. [35] have previously shown that the substrate templates the formation of flat crystallites of TIPS-pentacene with lamellar packing at the solid–liquid interface in the case of drop-casting experiments. A combination of in situ high-speed optical and μGIWAXS observations of the solution-shearing process in the current study supported the conclusion that the thin film crystallizes from the air–liquid interface, rather than from the solid–liquid interface. Yet, the resulting films are lamellar in texture. It therefore appears that the air–liquid interface of a very thin liquid film acts as a high-quality template for lamellar crystallites nucleated because of high supersaturation at the air–liquid interface. The liquid–air interface may be flatter and less defective than the solid–liquid interface, as it is not subject to surface roughness or surface chemical variations. Our work is supported by previous GIWAXS studies of blow drying of P3HT solutions, which showed that polymer crystallization occurred first at the air–liquid interface in conditions of rapid solvent evaporation [40] . For films where both the equilibrium and metastable polymorphs are present, the sequence of crystallization of the equilibrium and metastable polymorphs is very unusual, because it contradicts Ostwald’s rule of stages. The latter predicts that the metastable polymorphs should form first owing to a lower energy barrier and subsequently transform into the most stable phase potentially after transforming through one or more metastable polymorphs with progressively lower energy states [4] . We have recently demonstrated the polymorphism sequence in small-molecule solution-processable bulk heterojunction solar cells prepared by spin coating to be in agreement with Ostwald’s rule of stages [36] . The initially formed structure gradually transformed into the equilibrium structure in the presence of a solvent additive within the first minute of the spin-coating process. The deviation from the Ostwald rule of stages points to important differences between the crystallization behaviour of small-molecule thin films prepared by spin coating and solution shearing. A major difference we see thus far from the evidence at hand is that crystallization is initiated at the liquid–air interface in the solution-shearing process as opposed to the solid–liquid interface, which is where crystallization of small molecules is initiated in drop- and spin-casting processes [35] . When crystallization is initiated at the surface of the solution and proceeds towards the substrate, it confines the solution in one dimension, thereby forcing crystallization to occur in a confined space. This is analogous, we believe, to the crystallization of organic compounds in nanoporous media. Crystallization of pharmaceutical compounds in nanoscale pores has been shown to enable selective crystallization of different polymorphs [38] , [41] . We observed that the solvent molar volume allowed us to control the extent of metastable polymorph formation. Specifically, increasing the molar volume of the solvent resulted in a larger displacement from the equilibrium polymorph for a wide range of solvents. The observed correlation between the solvent molar volume and polymorphism is a remarkable and surprising result. We first explored the most obvious solvent parameters, such as the film thickness, shearing temperature, the boiling point, the solubility or Hansen parameters, but we could not find any meaningful correlation with these parameters ( Supplementary Fig. 7 and Supplementary Table 1 ). For instance, tetralin, which has the highest boiling point among the solvents explored, required a higher temperature ( T =174 °C), yet it showed a smaller fraction of the metastable polymorph as compared with mesitylene, which was sheared at a lower temperature ( T =125 °C) ( Supplementary Fig. 8 ). We also exclude the possibility of non-covalent chemical interactions between the OSC and solvent being the cause for polymorphism. Hansen parameters, which take such interactions into account, did not correlate with the degree of peak shift from the equilibrium position ( Supplementary Table 1 ). The solubility of TIPS-pentacene in the various solvents at the shearing temperatures used is also relatively high (>200 mg ml −1 for tetrahydrofuran, toluene, dicholorobenzene, mesitylene and decalin), thus precluding solubility as a key contributing factor for the observed differences in peak position shift. Finally, one may try to relate the formation of metastable polymorphs to the shear field generated during solution shearing [42] . The shear rates caused by the top plate moving at 1 mm s −1 and a gap of 100 μm is ~10 s −1 , so it is unlikely that high shear rates caused by the motion of the top plate are responsible for the metastable polymorph formation. However, surface tension gradient driven flows can cause high shear rates near the drying line [43] . In pure liquid crystals, shear rates on the order of 10 s −1 can produce non-equilibrium structures as well [44] . It has also been shown that both confinement and shear can give rise to polymorphism in liquid crystals [45] , [46] . Therefore, it is possible that the combined kinetic effects of shear and solvent drying, as well as confinement effects during solution shearing may generate TIPS-pentacene polymorphs. Having explored the most obvious parameters without finding any meaningful correlations, we turned to a consideration of the molar volume and the surface tension of the solvents in question. According to the Eötvös rule, the surface tension of a solvent at any shearing temperature is proportional to ( T c − T )/( V m 2/3 ), where T c is the critical temperature of the solvent, T is the shearing temperature and V m is the molar volume. The surface tension of the solvents generally decreases with increasing molar volume at our shearing temperatures, as shown in Fig. 6a . It is possible for the solvent surface energy to alter the Gibbs free energy of the system in a manner that modifies the polymorphic outcome of the solution-shearing experiment. The molecular size of the solvent may also have a kinetic effect as it may require a larger displacement or conformational change by the OSC molecule before incorporating into the crystal facet. For instance, decalin—the solvent with the largest molar volume (256 Å 3 per molecule)–has nearly half the molecules in the confinement space and half the molecules per solute molecule as compared with tetrahydrofuran, the solvent with the smallest molar volume (134 Å 3 per molecule) among those tested. We used molecular simulation techniques to determine the effect of solvent molecule size (in terms of the molar volume) on the energetic preference for a particular polymorph of the TIPS-pentacene ( Supplementary Figs 9 and 10 ; Supplementary Tables 2 and 3 ). Increasing solvent size is found to destabilize the configurational stability of the TIPS-pentacene unit cell ( Fig. 6b ). Although these simulations do not capture the effect of the solvent molecule in the bulk liquid phase as the unit cell is forming, they do point to the intriguing role played by solvent molar volume in mediating polymorphism, independent of other parameters such as process temperature and polar effects [47] . It is possible, but purely speculative at this stage, whether a molecular-scale process associated with the mass transport of solvent and solute molecules during the rapid crystallization process may be responsible for promoting the observed polymorphism. The uncertain nature of these two explanations should take nothing away from the remarkable and demonstrated ability to tune polymorphism via solvent selection in the solution-shearing process. Further studies need to be performed, both experimental and computational in nature, to shed more light into the mechanistic background of the results reported herein. 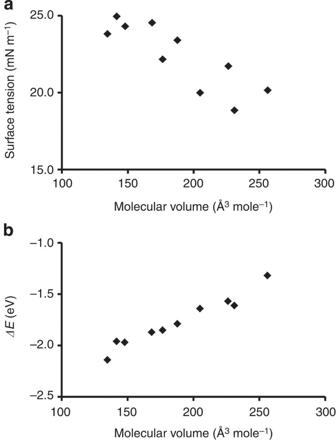Figure 6: Effect of solvent surface tension and molecular size on metastable polymorphism. (a) Relationship of the surface tension and molecular volume of the different solvents at their respective shearing temperatures, as obtained from the Eötvös equation. The shearing temperature was adjusted to achieve the same evaporation rate for all solvents. (b) Lennard–Jones ‘solvents’ and their effect on the energetics of preferred crystal structure parameters. Figure 6: Effect of solvent surface tension and molecular size on metastable polymorphism. ( a ) Relationship of the surface tension and molecular volume of the different solvents at their respective shearing temperatures, as obtained from the Eötvös equation. The shearing temperature was adjusted to achieve the same evaporation rate for all solvents. ( b ) Lennard–Jones ‘solvents’ and their effect on the energetics of preferred crystal structure parameters. Full size image In conclusion, we investigate the formation of metastable polymorphs of TIPS-pentacene during the solution-shearing process. This is accomplished by applying high-speed in situ μGIWAXS and in situ POM techniques that allow us to observe the crystallization sequence on a timescale of milliseconds. Time-resolved and static GIWAXS measurements support the conclusion that nucleation occurs from the liquid–air interface, thus forming a crust at the surface of the solution that self-confines the crystallization front along the vertical direction. The resulting films exhibit remarkably good lamellar texturing despite the crystallization not being templated from the solid–liquid interface as in other solution processes. Importantly, we show that vertical self-confinement can promote metastable polymorphism in a manner analogous to what 3D nanoscale confinement has been shown to do in the pharmaceutical industry. By changing the concentration of the solution, we vary the thickness of the film and achieve different degrees of self-confinement of the crystallization front that allow us to enhance or attenuate the polymorphism we seek, and thus verify the confinement hypothesis. We further demonstrate that the use of solvents with larger molar volume and by extension of lower surface tension more readily promotes the effects of confinement and results in metastable polymorphism. These findings allow us to better identify the solution-processing conditions needed to promote the formation of metastable polymorphs of OSCs over large areas, and to tune the electronic structure of the resulting polycrystalline OSC films for a variety of applications. Looking beyond organic electronics, the solution-shearing approach should also be a promising method to control crystal polymorphism in the pharmaceutical industry and beyond. Materials The TIPS-pentacene (received from Sigma-Aldrich Co.) was used without further purification. Phenyltrichlorosilane (PTS) and n -octadecyltrimethoxysilane (OTS) were purchased from the Sigma-Aldrich Co. and used as received (storage under an Argon atmosphere after the containers were opened to prevent hydrolysis). Silicon wafers with either a 300-nm thermally grown silicon oxide or a native oxide layer were used as the substrates for thin-film fabrication, as well as for static and time-resolved GIWAXS. Substrate preparation and characterization The silicon wafers were cleaned in a Piranha solution (70/30 v/v H 2 SO 4 /H 2 O 2 ; caution: highly oxidative solution, violent reaction may take place when in contact with organic materials) for 25 min. The bottom thin-film substrate (1.5 × 1.5 cm 2 ) was treated with PTS to ensure proper wetting for the TIPS-pentacene solution. PTS treatment was accomplished by immersing the Piranha-cleaned wafer into a toluene solution of PTS (3 wt%) and heated at 90 °C for 15 h. The substrate was subsequently removed from PTS solution and was sonicated for 2 min in toluene. It was then gently wiped with a sponge tip and rinsed sequentially with toluene, acetone and isopropanol. The water contact angle of the PTS-treated surface ranged from 75° to 79°. The typical roughness (root mean squared, r.m.s.) of the surface was 0.3–0.5 nm, as measured by atomic force microscopy. For the top shearing plate, a silicon wafer with a 300-nm thermally grown oxide was treated with a monolayer of OTS according to a method we published previously for forming a highly hydrophobic crystalline OTS monolayer [22] , [30] . The OTS treatment is important to ensuring deposition of TIPS-pentacene only on the bottom PTS-treated substrate. The water contact angle of the OTS-modified surface ranged between 102° and 104°, and the r.m.s. surface roughness ranged between 0.2 and 0.5 nm. Solution shearing of TIPS-pentacene films The TIPS-pentacene solution was prepared at a concentration of 4, 8 or 16 mg ml −1 in various solvents listed in Supplementary Table 1 and in previous work [5] . Both the device substrate and the shearing plate were held in place by respective vacuum chucks while the substrate was mounted on a resistively heated stage (a thermoelectric module from Custom Thermoelectric Co.). After placing ~10 μl cm −2 of TIPS-pentacene solution on the device substrate, the shearing plate was lowered with a micromanipulator to make contact with the solution. The device substrate was horizontal while the shearing plate was placed at a tilt angle of 8 degrees from horizontal. The gap distance between the device substrate and the shearing plate was fixed at 100 μm. The shearing plate was moved at different velocities by a microstepping translation stage. The resulting sheared film was left on the heating stage for 2–3 min to remove residual solvent. Characterization of solution sheared thin films Static GIWAXS was performed at the Stanford Synchrotron Radiation Lightsource on beamline 11-3. A photon energy of 12.73 keV was used and the scattering intensity was recorded on a 2D image plate (MAR-345) with a pixel size of 150 μm (2,300 × 2,300 pixels) located at a distance of 400 mm from the sample centre. The distance between the sample and the detector was calibrated using a LaB 6 polycrystalline standard. The incidence angle was chosen in the range of 0.04°–0.14°. The beam size was 50 μm × 150 μm that resulted in a beam exposure on the sample 150 μm wide over the entire length of the 10 mm sample. The data was distortion corrected (theta-dependent image distortion introduced by planar detector surface) before performing quantitative analysis on the images. Numerical integration of the diffraction peak areas was performed with the software WxDiff. The overall resolution in the GIWAXS experiments, dominated by the sample size, was about 0.02 Å −1 . In situ GIWAXS Static and in situ time-resolved microbeam μGIWAXS measurements were performed at CHESS on D-line. The X-ray beam with a wavelength of 1.15 Å and with a wide bandwidth of 1.5% was focused to a beam size of 15 × 15 μm 2 using a single-bounce X-ray focusing capillary. The sample was placed in the focal point, 55 mm away from the end of the capillary. The incidence angle was chosen as 0.15°. The blade was aligned parallel to the beam footprint using a camera located on the top of the sample. The scattering intensity was recorded at a speed of up to 100 frames per second using a Pilatus 100 K area detector with a pixel size of 172 μm at a distance of 195 mm from the sample centre. The rectangular detector was placed 40 mm off the reflection plane in an upright orientation to record the relevant in-plane diffraction peaks during the casting process. In situ high-speed POM High-speed POM was performed at KAUST on a Nikon LV100 microscope and recorded by a Photron SA-3 CMOS camera. The camera was mounted on the microscope with a fixed angle of 75° between polarizer and analyser. The images were recorded at a speed of 125 frames per second with a shutter speed of 0.004 s. How to cite this article: Giri, G. et al. One-dimensional self-confinement promotes polymorph selection in large-area organic semiconductor thin films. Nat. Commun. 5:3573 doi: 10.1038/ncomms4573 (2014).